Refractory dissolved organic nitrogen accumulation in high-elevation lakes The role of dissolved organic matter (DOM) as either a sink for inorganic nutrients or an additional nutrient source is an often-neglected component of nutrient budgets in aquatic environments. Here, we examined the role of DOM in reactive nitrogen (N) storage in Sierra Nevada (California, USA) lakes where atmospheric deposition of N has shifted the lakes toward seasonal phosphorus (P)-limitation. Nuclear magnetic resonance (NMR) spectroscopy and isotope analyses performed on DOM isolated from Lake Tahoe reveal the accumulation of refractory proteinaceous material with a 100–200-year residence time. In contrast, smaller lakes in the same watershed contain DOM with typical terrestrial characteristics, indicating that proteins in Lake Tahoe are autochthonously produced. These data support the role of DOM as a possible sink for reactive N in these lake ecosystems and identify a potential role for DOM in affecting the inorganic nutrient stoichiometry of these environments. Widespread atmospheric N deposition on nutrient-limited aquatic environments has begun to alter primary production and community composition [1] , and the nutrient inventories of remote lakes are being perturbed by growing inputs of N from the atmosphere [2] . It has been demonstrated that lake ecosystems may compensate for nutrient imbalance by altering phytoplankton communities [3] . Other ecosystem processes, including sedimentary denitrification [4] , that remove reactive N could also enable lacustrine microbial food webs to modulate lake N:P stoichiometry. The pool of dissolved organic matter (DOM) is an important currency of energy and nutrient exchange within and between terrestrial ecosystems, including aquatic environments [5] . Several recent studies have shown that lakes are important sites of terrestrial organic carbon degradation and thus, net CO 2 production [6] , [7] , [8] . The intermittent storage of reactive N within lake-dissolved organic nitrogen (DON), including seasonal enrichment of protein-like fluorescence, has also been reported and attributed to recent primary and secondary production [9] , [10] . These examples highlight the role of DOM in lake carbon (C) and nutrient biogeochemistry, yet this reservoir is rarely considered in modelling efforts that interrogate the response of lake ecosystems to change. Pristine, oligotrophic, high-elevation lakes are recognized as sentinels of change due to their heightened sensitivity to climatic variations and eutrophication [11] . This makes them appropriate environments in which to examine lake biogeochemistry, including DOM cycling, which plays a critical role in energy transfer and in nutrient cycling in these environments. In this study, the contribution of autochthonous and allochthonous processes to C and N storage within DOM was examined in the Lake Tahoe Basin, which is a high-elevation watershed in the California Sierra Nevada. Lake Tahoe (LT) is the largest lake within this watershed, and climate change and atmospheric N deposition have already begun to alter its phytoplankton species composition and nutrient stoichiometry [12] , [13] , [14] , [15] , [16] . There are several lakes in this basin that share similar external C and N inputs, but they vary widely in size and water residence time. This sets up an ideal experimental system for examining the role of the lacustrine reactor in determining residence time and speciation of nutrients. The specific study design incorporated lakes with short (Upper Angora Lake; UAL), mid-range (Fallen Leaf Lake; FLL) and long (LT) water residence times that were sampled during periods of both high and low inflow. The very short water residence time of UAL should enable the characteristics of allochthonous DOM and nutrient inputs to be examined in isolation, while LT’s 300–650 year residence time facilitates the detection of any allochthonous and autochthonous DOM that accumulates on long time scales in these lakes. A suite of DOM isotopic and chemical composition measurements reveals significant differences between UAL and LT, and supports the hypothesis that terrestrial compounds are most prevalent in the smallest lake, which also has the shortest hydraulic residence time. Marked temporal variability exists in FLL, with some samples exhibiting chemical characteristics previously attributed to long-lived DOM [17] , [18] . In LT, we detect the long-term accumulation of dissolved proteins, and the isotopic signature of the N-rich DOM fraction points to in-lake conversion of reactive N to refractory proteins. Our study examines three geographically restricted lakes; however, on the basis of findings described here, previous reports of seasonal DON production in lakes around the world [7] , [9] , [10] , [19] suggests that the identical phenomenon of reactive N partitioning into dissolved proteins could occur globally. Dissolved organic carbon at lake study sites Samples were collected seasonally for dissolved organic carbon (DOC) at all sites ( Fig. 1 ; Supplementary Fig. 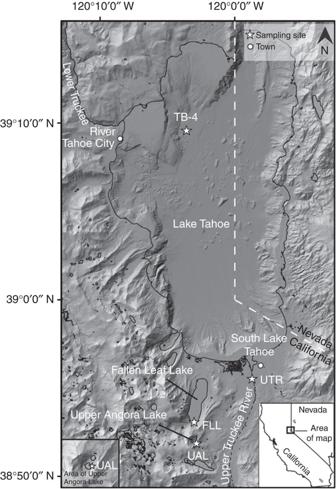Figure 1: Map of Lake Tahoe Basin in the area of California and Nevada. The sampling sites were Lake Tahoe (LT; TB-4), Fallen Leaf Lake (FLL), Upper Angora Lake (UAL; see inset in lower left corner) and the Upper Truckee River (UTR). The UTR is not drawn to scale. Because of the small size of UAL on the main map, the inset is provided to magnify (three times relative to the main map) the area surrounding UAL to show this sampling location in finer detail. The image was downloaded from the United States Geological Survey (USGS) website (http://tahoe.usgs.gov/DEM.html). 1 and Table 1 ). Concentrations of DOC in UAL and the upper truckee river (UTR) were 111 to 136 μmol C l −1 , 3- to 4-fold higher than LT ( Table 1 ). The lowest concentrations of DOC were observed in LT and were comparable to previous work [20] . Surface concentrations varied by ~10 μmol C l −1 in LT over the three time points ( Table 1 ), but relatively stable concentrations (~28 μmol C l −1 ) were observed below ~150 m ( Supplementary Fig. 2 ). Fallen Leaf Lake showed intermediate concentrations of 73–79 μmol C l −1 . Figure 1: Map of Lake Tahoe Basin in the area of California and Nevada. The sampling sites were Lake Tahoe (LT; TB-4), Fallen Leaf Lake (FLL), Upper Angora Lake (UAL; see inset in lower left corner) and the Upper Truckee River (UTR). The UTR is not drawn to scale. Because of the small size of UAL on the main map, the inset is provided to magnify (three times relative to the main map) the area surrounding UAL to show this sampling location in finer detail. The image was downloaded from the United States Geological Survey (USGS) website ( http://tahoe.usgs.gov/DEM.html ). Full size image Table 1 Mean molar C:N and isotopic characteristics of SPE-DOM from Lake Tahoe Basin sampling sites. Full size table Extracted DOM elemental and isotope signatures The per cent recovery of DOC following solid-phase extraction (SPE) and elution was 10–35%, with LT samples generally having higher recoveries ( Table 1 ). Carbon recovery reported in Table 1 was calculated on the basis of the DOC eluted from the DAX-8 column using the specified solvent. For the terrestrial-type samples from UAL and UTR, DOC recoveries estimated from determining the DOC concentration of the column permeate were comparable to other work [21] (see Supplementary Methods on reporting recovery efficiencies). The bulk chemical characteristics observed in LT SPE-DOM are unique from UAL and UTR ( Table 1 and Fig. 2 ). Upper Angora and UTR SPE-DOM samples exhibit terrestrial characteristics; they are low in δ 13 C and δ 15 N (−26.0 to −26.8‰ and 0.7 to 1.6‰, respectively) and have high C:N ratios (33.3 to 38.8). In contrast, LT SPE-DOM is more enriched in δ 13 C and δ 15 N (−19.8 to −17.7‰ and 4.9 to 5.3‰, respectively) and has low C:N ratios (3.7 to 4.5). The SPE-DOM from FLL appears to oscillate between the chemical characteristics of LT and of the terrestrial endmembers UAL and UTR, indicating it is sensitive to seasonally varying DOM sources and sinks. As all lake-water samples were identically processed across sites and seasons, the unique chemical characteristics observed for LT must reflect real differences between lakes in the composition of their bulk DOM rather than artifacts of sample processing. Also, the C:N ratio of extracted DOM, which is a proxy for the composition of DOM in this case, was not significantly correlated with recoveries ( P =0.091). 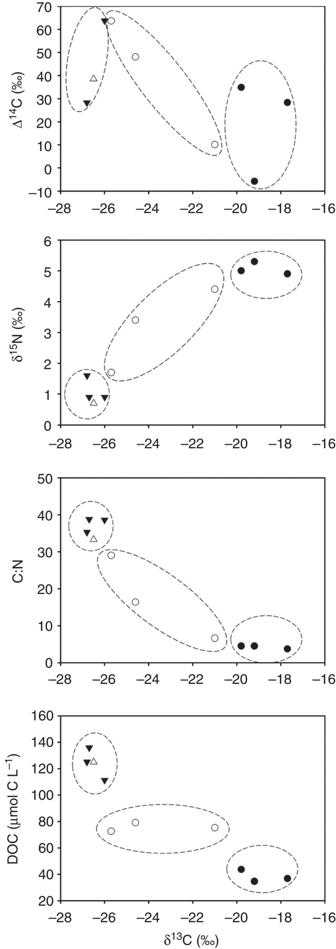Figure 2: Seasonal variability of dissolved organic matter elemental and isotopic composition. The stable carbon isotope signature (δ13C in per million; ‰) of solid-phase extracted dissolved organic matter (SPE-DOM) differentiates autochthonous endmembers, such as SPE-DOM from Lake Tahoe (LT; closed circles) and Fallen Leaf Lake (FLL; open circles), from the terrestrially influenced SPE-DOM samples of Upper Angora Lake (UAL; closed triangles) and the Upper Truckee River (UTR; open triangle). The SPE-DOM samples separated in this manner also exhibit unique radiocarbon signatures (Δ14C in ‰;n=9), elemental compositions (C:N;n=10) and stable nitrogen isotope signatures (δ15N in ‰;n=10). The total dissolved organic carbon (DOC) concentrations (μmol C l−1;n=10) measured at the time of SPE-DOM collection also appear to be lake specific. The greatest seasonal variability is detected in FLL, where allochthonous, terrestrial characteristics are detected in SPE-DOM during periods of high inflow in spring/early summer. Ellipses serve to more clearly differentiate samples from one another. Figure 2: Seasonal variability of dissolved organic matter elemental and isotopic composition. The stable carbon isotope signature (δ 13 C in per million; ‰) of solid-phase extracted dissolved organic matter (SPE-DOM) differentiates autochthonous endmembers, such as SPE-DOM from Lake Tahoe (LT; closed circles) and Fallen Leaf Lake (FLL; open circles), from the terrestrially influenced SPE-DOM samples of Upper Angora Lake (UAL; closed triangles) and the Upper Truckee River (UTR; open triangle). The SPE-DOM samples separated in this manner also exhibit unique radiocarbon signatures (Δ 14 C in ‰; n =9), elemental compositions (C:N; n =10) and stable nitrogen isotope signatures (δ 15 N in ‰; n =10). The total dissolved organic carbon (DOC) concentrations (μmol C l −1 ; n =10) measured at the time of SPE-DOM collection also appear to be lake specific. The greatest seasonal variability is detected in FLL, where allochthonous, terrestrial characteristics are detected in SPE-DOM during periods of high inflow in spring/early summer. Ellipses serve to more clearly differentiate samples from one another. Full size image NMR spectroscopy Proton ( 1 H) NMR spectra of SPE-DOM isolated from LT in June 2010 and FLL in August 2009 are unusual for DOM. They show better-defined peaks than the unresolved humps that are typical for DOM [22] and observed for UAL ( Fig. 3 ) and UTR ( Supplementary Figs 3 and 4 ). Prominent resonances in the 0.8–1.4, 1.5–1.8, 1.8–3.2 and 3.4–4.8 p.p.m. regions of the 1 H NMR spectrum ( Fig. 3 and Supplementary Fig. 3 and Fig. 4b ) and discernible features in the aromatic region (6.5–8.0 p.p.m. ; Fig. 3 and Supplementary Fig. 4c ) differentiate these samples from typical DOM. Closer inspection reveals that many of these largest peaks are consistent with protein resonances [23] , [24] . 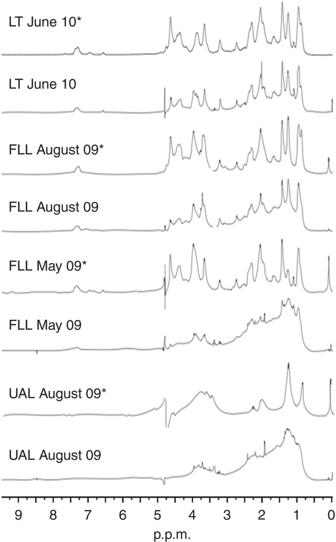Figure 3: Nuclear magnetic resonance spectra for dissolved organic matter. The spectra reveal chemical functional group variability across lakes. A comparison of the diffusion-edited (denoted by *) spectrum with the original spectrum reveals that macromolecular/rigid proteins dominate the proton nuclear magnetic resonance (1H NMR) spectrum of solid-phase extracted dissolved organic matter (SPE-DOM) from Lake Tahoe (LT) and Fallen Leaf Lake (FLL) in August 2009 (August 09). All resonances in the spectrum are consistent with proteins, where resonances in the 3.4–4.5 p.p.m. region are particularly characteristic of the α-C-H group of amino acids. In contrast, the NMR spectrum for SPE-DOM isolated from FLL in May 2009 (May 09) contains resonances more typical of terrestrial SPE-DOM that are also found in Upper Angora Lake (UAL). These spectra contain enhanced contributions from lipid resonances (0.8–2.5 p.p.m.). However, the diffusion-edited spectrum confirms that macromolecular DOM in FLL May 09 is compositionally similar to the protein-like functional groups identified in LT and FLL August 09. These data further reveal that dissolved proteins likely accumulate in FLL throughout the year, but are masked by terrestrial inputs and dominated by smaller molecules during the spring season. Finally, the diffusion-edited NMR spectrum for UAL is unique in this sample set. A comparison between the diffusion-edited and original spectrum indicates that many of the lipid resonances present in UAL SPE-DOM are associated with smaller/faster diffusing structures, and that macromolecular/rigid terrestrial DOM is dominated by resonances that are also present in carbohydrates (3–4 p.p.m.). Figure 3: Nuclear magnetic resonance spectra for dissolved organic matter. The spectra reveal chemical functional group variability across lakes. A comparison of the diffusion-edited (denoted by *) spectrum with the original spectrum reveals that macromolecular/rigid proteins dominate the proton nuclear magnetic resonance ( 1 H NMR) spectrum of solid-phase extracted dissolved organic matter (SPE-DOM) from Lake Tahoe (LT) and Fallen Leaf Lake (FLL) in August 2009 (August 09). All resonances in the spectrum are consistent with proteins, where resonances in the 3.4–4.5 p.p.m. region are particularly characteristic of the α-C-H group of amino acids. In contrast, the NMR spectrum for SPE-DOM isolated from FLL in May 2009 (May 09) contains resonances more typical of terrestrial SPE-DOM that are also found in Upper Angora Lake (UAL). These spectra contain enhanced contributions from lipid resonances (0.8–2.5 p.p.m.). However, the diffusion-edited spectrum confirms that macromolecular DOM in FLL May 09 is compositionally similar to the protein-like functional groups identified in LT and FLL August 09. These data further reveal that dissolved proteins likely accumulate in FLL throughout the year, but are masked by terrestrial inputs and dominated by smaller molecules during the spring season. Finally, the diffusion-edited NMR spectrum for UAL is unique in this sample set. A comparison between the diffusion-edited and original spectrum indicates that many of the lipid resonances present in UAL SPE-DOM are associated with smaller/faster diffusing structures, and that macromolecular/rigid terrestrial DOM is dominated by resonances that are also present in carbohydrates (3–4 p.p.m.). 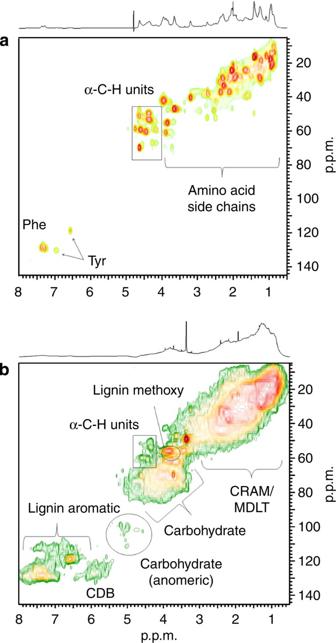Figure 4: Nuclear magnetic resonance-assigned biochemical classes in lake-dissolved organic matter. Heteronuclear Single Quantum Coherence (HSQC) nuclear magnetic resonance (NMR) spectra for lake samples with autochthonous (Lake Tahoe) and allochthonous (Upper Angora Lake) endmember characteristics enable assignment of broad chemical classes to the solid-phase extracted dissolved organic matter (SPE-DOM) present in each sample. The proton (1H) NMR spectrum and its scale (xaxis in p.p.m.) are shown at the top and bottom of each panel, respectively, for (a) Lake Tahoe and (b) Upper Angora Lake. Theyaxis is the carbon (13C) NMR scale (in p.p.m.). Contours and colours represent the abundance of particular resonances where red is most abundant and green is least abundant. The dominance of proteins in Lake Tahoe SPE-DOM is apparent in the intensity of NMR resonances associated with amino-acid side chains from 0 to 3.4 p.p.m. (1H resonances,xaxis) and 10 to 60 p.p.m. (13C resonances,yaxis), protons located on carbon atoms alpha to the peptide bond (α-C-H), and the individual amino acids phenylalanine (Phe) and tyrosine (Tyr). The respective 0–3.4 p.p.m.1H NMR and 10–60 p.p.m.13C NMR regions for the Upper Angora Lake sample lack the protein signature, and are instead dominated by carboxyl-rich alicyclic molecules (CRAM) and material derived from linear terpenoids (MDLT) as defined in refs17,18The added presence of resonances from lignin methoxy groups, conjugated double bonds (CDBs), α-C-H units, lignin aromatics, carbohydrates and protons on the anomeric carbon of carbohydrates are also defined in the Upper Angora Lake spectrum, and further delineate differences between this allochthonous sample and Lake Tahoe. Full size image Figure 4: Nuclear magnetic resonance-assigned biochemical classes in lake-dissolved organic matter. Heteronuclear Single Quantum Coherence (HSQC) nuclear magnetic resonance (NMR) spectra for lake samples with autochthonous (Lake Tahoe) and allochthonous (Upper Angora Lake) endmember characteristics enable assignment of broad chemical classes to the solid-phase extracted dissolved organic matter (SPE-DOM) present in each sample. The proton ( 1 H) NMR spectrum and its scale ( x axis in p.p.m.) are shown at the top and bottom of each panel, respectively, for ( a ) Lake Tahoe and ( b ) Upper Angora Lake. The y axis is the carbon ( 13 C) NMR scale (in p.p.m.). Contours and colours represent the abundance of particular resonances where red is most abundant and green is least abundant. The dominance of proteins in Lake Tahoe SPE-DOM is apparent in the intensity of NMR resonances associated with amino-acid side chains from 0 to 3.4 p.p.m. ( 1 H resonances, x axis) and 10 to 60 p.p.m. ( 13 C resonances, y axis), protons located on carbon atoms alpha to the peptide bond (α-C-H), and the individual amino acids phenylalanine (Phe) and tyrosine (Tyr). The respective 0–3.4 p.p.m. 1 H NMR and 10–60 p.p.m. 13 C NMR regions for the Upper Angora Lake sample lack the protein signature, and are instead dominated by carboxyl-rich alicyclic molecules (CRAM) and material derived from linear terpenoids (MDLT) as defined in refs [17] , [18] The added presence of resonances from lignin methoxy groups, conjugated double bonds (CDBs), α-C-H units, lignin aromatics, carbohydrates and protons on the anomeric carbon of carbohydrates are also defined in the Upper Angora Lake spectrum, and further delineate differences between this allochthonous sample and Lake Tahoe. Full size image Resonances consistent with proteins (0–4.5 p.p.m.) can be emphasized by the use of diffusion editing ( Fig. 3 ), which typically suppresses resonances derived from compounds not incorporated into macromolecular/rigid domains [25] (see Supplementary Discussion and Supplementary Methods for details). Dominant resonances in DOM from LT in June 2010 and FLL in August 2009 are barely affected by diffusion editing, indicating that they are of a true macromolecular origin. Diffusion editing reveals the same protein-like profile in FLL in May 2009 ( Fig. 3 ). Without diffusion editing, these resonances in FLL May 2009 are masked by complex signals between 0–4.5 p.p.m. In contrast, the diffusion-edited spectrum from UAL contains no clear signals from protein ( Fig. 3 ). The spectral profile of the slowly diffusing macromolecules within the UAL sample is more consistent with larger aliphatic materials and carbohydrates ( Fig. 3 ). Conclusive assignment of resonances in LT samples was performed via two-dimensional (2D) NMR. The 1 H– 13 C heteronuclear Single Quantum Coherence (HSQC) spectrum ( Fig. 4a ) clearly identifies the majority of peaks to be consistent with protein [26] , [27] . This is particularly evident for the protein α-C-H region (3.4–4.5 p.p.m.) in the HSQC spectrum, which is completely resolved owing to the high protein content of the sample ( Fig. 4a ). These resonances have similar spectral characteristics in FLL SPE-DOM from May and August ( Fig. 3 ). Utilizing the prominence of these resonances in LT SPE-DOM, saturation transfer difference (STD) NMR spectroscopy was used to differentiate between other resonances belonging to protein from those that belong to unrelated compound classes ( Supplementary Fig. 5 ; see Supplementary Discussion and Supplementary Methods ). A comparison between the diffusion-edited ( Supplementary Fig. 5b ) and STD spectra ( Supplementary Fig. 5c ) indicates that all major signals in LT arise from protein. Line-shape estimations reveal that the protein signal envelope dominates the entire spectral profile and accounts for ~90% of the total NMR signal of LT SPE-DOM. When considering FLL SPE-DOM from May in which diffusion editing revealed a mixture of protein and other more complex resonances, STD spectroscopy enabled an estimation of the relative protein content. Linear combination of ‘terrestrial-like’ SPE-DOM from UAL and autochthonous ‘protein-like’ SPE-DOM from LT estimated that each of these NMR ‘spectral’ types contributed ~50% to the spectral envelope of the FLL May sample. Traces of protein may be present in the UAL sample, as indicated by highlighted resonances that appear in the α-C-H functional group region of the HSQC spectrum. However, line-shape estimation revealed that proteins represented <5% of the total UAL NMR profile. Molecular indices of terrestrial input Lower lignin–phenol concentrations (Σ 8 ; Supplementary Table 2 ) corresponded to more positive δ 13 C values ( Supplementary Fig. 6 ), and together these proxies point to the diminished influence of recent terrestrial OM inputs to LT and FLL August SPE-DOM. Enriched δ 13 C signatures of these latter samples must instead identify a dominant autochthonous DOM contribution. Δ 14 C of SPE-DOM and DIC and δ 13 C of DIC The SPE-DOM samples isolated from UAL, UTR and FLL (May, July) have Δ 14 C signatures ranging from 28 to 64‰ ( Table 1 ). This is similar to the Δ 14 C of atmospheric CO 2 in the Northern Hemisphere in 2009–2010 (for example, 45‰) [28] . The SPE-DOM isolated from FLL in August and LT in May 2009 and June 2010 have Δ 14 C signatures ranging between 10 and 35‰, at the lower end of the range observed in UTR, UAL and FLL (May, July; Table 1 ). However, the Δ 14 C signature of surface SPE-DOM in LT during January 2010, −6‰, was significantly depleted in 14 C relative to all other values. In contrast, Δ 14 C of dissolved inorganic carbon (DIC) in LT was significantly more enriched: ~110‰ at the surface and ~128‰ at 440 m ( Table 1 ). The highest δ 13 C value for DIC of lake water was observed in surface LT (+0.4‰), and the lowest value was observed in UAL (−10.1‰; Table 1 ). Intermediate values were measured for DIC from deep LT (−0.8‰) and FLL (−2.2‰). All of these measurements were made during June/July 2010, and depleted δ 13 C-DIC in UAL is consistent with a DIC contribution from respired allochthonous organic C. Radiocarbon model for Lake Tahoe The Δ 14 C signatures of DIC and DOC were used to estimate their turnover time scales with a simple box model framework. Dissolved inorganic carbon and DOC in LT were assumed to be two single, well-mixed reservoirs of carbon [29] . In the model, Δ 14 C-DIC in LT responds to transient changes in Δ 14 C of atmospheric CO 2 observed in the Northern Hemisphere [30] through air–lake exchange. Changes in atmospheric Δ 14 C are propagated to DIC and then to DOC according to the turnover time scales of each reservoir (in equation 1 τ DIC and τ DOC ; see the Supplementary Discussion for further details on these assumptions). According to this simple framework, the tendencies of Δ 14 C of DIC and DOC follow the equations: where R DIC and R DOC indicate the normalized 14 C/C ratio (that is, Δ 14 C/1,000‰+1) in DIC and DOC. The R A term indicates the corresponding ratio in Northern Hemisphere atmospheric CO 2 , which was specified using atmospheric observations [30] , [31] , [32] . Radioactive decay of 14 C with a mean life of 5,730/ln 2 (for example, 8,267 years) is also included in the model. The production and respiration of DOC was assumed to have no effect on DIC because the concentration of DOC (28–44 μmol C l −1 ) is much lower than DIC (900–960 μmol C l −1 ). The DOC in the model is purely autochthonous. Elevated Δ 14 C in deep water DIC (128‰) compared with atmospheric Δ 14 C (45‰) in 2009–10 is indicative of a decadal time scale for DIC turnover in LT since atmospheric Δ 14 C levels were much higher in previous decades because of 14 C production by nuclear weapons testing [29] , [30] , [31] . Atmospheric Δ 14 C has decreased in a nearly exponential manner from a maximum value of >700‰ at the conclusion of large-scale nuclear weapons testing in the 1960s. Varying the model’s DIC turnover time scale (τ DIC ) to best fit observed Δ 14 C-DIC values yielded two potential matches for τ DIC : 13.5 and 60 years. τ DIC relates directly to the gas transfer velocity, which is commonly parameterized using wind speed. The 13.5-year time scale can be rejected because the corresponding gas transfer velocity is associated with a wind speed of 11 ms −1 (ref. 33 ), which is much higher than observed at LT. The 60-year time scale corresponds to a mean wind speed of 3 ms −1 , which is similar to the mean wind speed of 2 ms −1 over LT used by Alin et al. [34] The simulated temporal evolution of lake Δ 14 C-DIC, for the optimal turnover time scale in DIC of 60 years, was used to examine the turnover time scale of SPE-DOM ( Supplementary Fig. 7 ). The box model was constrained using SPE-DOM collected in May 2009 and Jan 2010 (Δ 14 C for SPE-DOM of ~28‰ and −6‰, respectively), which corresponded to the lowest surface water DOC concentrations measured during the study. Therefore, these Δ 14 C values for SPE-DOM should closely approximate the radiocarbon signature of background/refractory SPE-DOM in LT. To fit these measured values of 28‰ to −6‰, a 100–200-year residence time for SPE-DOM in LT is required. Radiocarbon mass balance for Lake Tahoe SPE-DOM Unlike the depleted Δ 14 C signature observed for LT SPE-DOM in January 2010, SPE-DOM isolated from the same location in both May 2009 and June 2010 have higher Δ 14 C signatures and more elevated DOC concentrations. It is hypothesized here that the enrichment is derived from the multiple processes that contribute DOC to surface waters of LT during spring and summer. To first demonstrate how mixing between endmembers could alter the concentration and isotopic character of DOC (see Supplementary Fig. 8 and Supplementary Discussion ), the January 2010 and June 2010 SPE-DOM from LT were compared. It is assumed that the increase in surface bulk DOC concentration from 34.6 to 43.6 μmol C l −1 between January and June 2010 ( Table 1 ) reflects the accumulation of new, autochthonous DOC, and that the SPE-DOC concentration changed proportionally to DOC concentration. The seasonal change in Δ 14 C of SPE-DOM can then be reproduced by a two-endmember mass balance (see Supplementary Discussion for details; Supplementary Table 3a ). The endmembers in this case are background SPE-DOM observed in January (34.6±3.4 μmol C l −1 and −6±5‰) and autochthonous DOM (9.0±4.2 μmol C l −1 and 110±5‰). The mixture of these two endmembers is calculated to yield a Δ 14 C value of 18±18‰ for LT surface-accumulated total SPE-DOM in June. The predicted Δ 14 C value for SPE-DOM agrees with the measured value of 35‰, when the uncertainty of the measurements is considered. Small discrepancies are reasonable given that SPE-DOC concentrations are poorly constrained. This calculation neglects any terrestrial component of lake DOM even though there was a small increase in total lignin concentration in LT from January to June 2010 ( Supplementary Table 2 ). A three endmember model (see Supplementary Discussion ; Supplementary Table 3b ) that includes terrestrial DOM with Δ 14 C similar to atmospheric values (45‰) was tested and does not significantly change the correspondence to the observations (14.5±16‰ calculated versus 35‰ measured). According to radiocarbon constraints used in this mass balance, as much as 27% of fresh DOC input could be derived from terrestrial DOM. Overall, these endmember models can reproduce the observed seasonal variation in Δ 14 C by accounting for the stable concentration of background DOC in the deep waters of LT, annual lake mixing and seasonal autochthonous and allochthonous inputs of DOM ( Supplementary Fig. 8 ). Our examination of the DOM extracted onto DAX-8 resin from three Tahoe Basin lakes with varying water residence times, revealed the following: (1) proteins represent a significant fraction of the SPE-DOM in lakes with >1-year residence time; (2) these proteins appear to be autochthonous and to accumulate in LT on centennial time scales; (3) terrestrial SPE-DOM, in contrast, is mostly or entirely removed on annual time scales after entering these lakes; (4) the accumulation of autochthonous proteins could represent a newly recognized pathway for the removal of reactive nitrogen from lake systems. This study is the first to confirm the accumulation of a nearly pure protein fraction within DOM isolated from a lacustrine environment, accounting for ~30% of the DOC in LT based on SPE-DOM recoveries, C:N and NMR estimates that proteins account for >90% of the total NMR signal ( Table 1 ). The C:N of LT SPE-DOM ( Table 1 , Fig. 2 ) is lower than typical phytoplankton values (~6.7; ref. 35 ) and much lower than terrestrial organic matter (20–500; ref. 36 ). Instead, it is similar to that of cyanobacteria [37] , heterotrophic bacteria [38] and pure protein [39] . In addition, ~90% of the 1 H NMR resonances in LT SPE-DOM could be assigned to proteins. The diffusion-edited 1 H NMR spectrum ( Fig. 3 ) of LT SPE-DOM also confirms that these NMR resonances are present within macromolecules rather than either small peptides or other small molecules that contain amino-acid residues. These same protein NMR resonances are also detected in FLL, where they dominate the August 2009 sample and represent ~50% of proton resonances in the May 2009 sample ( Fig. 3 ). Protein 1 H NMR resonances have been previously identified in glacial [40] and lacustrine [41] DOM, and the presence of dissolved, fluorescent amino acids in subalpine lakes has been suggested via spectroscopic techniques [9] . Dissolved proteins could have sources throughout the watershed. For example, N-rich compounds can originate in soils due to selective preservation of refractory proteins [42] , [43] and/or production of labile proteins in situ [41] , [42] and then be transported via runoff and stream flow. Terrestrial DON can sometimes account for up to 90% of the N that enters high-elevation lakes [44] , [45] . However, accumulation of a protein-like fluorescence signal during warmer months has also been attributed to in situ production by lake microorganisms [9] , [19] , [46] , [47] . In contrast to the accumulation of dissolved proteins detected in LT and FLL, NMR experiments that were applied to UAL revealed the presence of larger aliphatic compounds, including ‘carboxy-rich alicyclic molecules’ and ‘molecules derived from linear terpenoids’, and carbohydrates ( Fig. 4b ) [17] , [18] . Similar compounds were also observed for SPE-DOM isolated from FLL May 2009 and July 2010 and the UTR ( Fig. 3 and Supplementary Fig. 3 ), and these compound classes have been previously described as typical of DOM [17] , [18] , [48] , [49] . The unique composition of SPE-DOM isolated from LT and FLL (August 2009), as compared with other shorter residence time lakes [7] , [10] , [47] , hints at an autochthonous rather than terrestrial source for accumulating proteins. The annual terrestrial DOC load entering LT can sustain the lake’s DOC inventory (see Supplementary Discussion and Supplementary Table 4 ), given its >300-year water residence time. However, SPE-DOM isotope and chemical composition data are inconsistent with the long-term accumulation of terrestrial SPE-DOM in LT. However, SPE does not isolate the entire pool of DOM, and the accumulation of terrestrial DOM, consisting of compounds other than those isolated from UAL and UTR, cannot be ruled out. On the basis of the data presented here, the combination of LT’s longer hydraulic residence time, lack of winter ice cover and high ultraviolet-transparency [50] , [51] likely allow for extensive bacterial degradation and photochemical alteration to impart a discernible DOM signature resulting from significant removal of some terrestrial compounds. For example, lignin–phenol concentrations in LT are similar to those measured in the open North Pacific Ocean [52] . Furthermore, the removal of allochthonous SPE-DOM by microbial and ultraviolet processing was evident in depleted δ 13 C-DIC values in FLL and UAL ( Table 1 ), which indicate DIC addition from organic matter degradation. Seasonal shifts in the chemical and isotopic composition of SPE-DOM due to terrestrial C delivery during snowmelt and its potential removal during late summer are most clearly illustrated in FLL. Chemical and isotopic characterization of SPE-DOM from May and July reveal chemical signatures typical of the terrestrial material listed above ( Table 1 ), including a relative enrichment in lignin oxidation products ( Supplementary Fig. 6 and Supplementary Table 2 ). In contrast, SPE-DOM isolated from FLL in August of 2009 was similar to LT samples with respect to elemental and isotope signatures ( Fig. 2 ), indicating that a significant fraction of incoming terrestrial DOM was removed over this time period. The 1 H NMR spectrum of the August 2009 SPE-DOM sample from FLL was also significantly altered relative to May 2009 and July 2010 samples. It is clear that this NMR spectrum has lost some significant resonances resembling carboxyl-rich alicyclic molecules, molecules derived from linear terpenoids and carbohydrate resonances common to the subset of terrestrial samples (UAL and UTR), and instead contains resonances primarily arising from proteins ( Fig. 3 ). This lake’s smaller volume relative to LT allows for the seasonal input of allochthonous DOM to dominate in the spring and early summer, while its longer residence time relative to UAL allows for autochthonous DOM to be detected. Similar seasonal transformations of DOM NMR resonances have been observed in other lake environments and attributed to microbial degradation [53] . However, photo-oxidation can also be an important pathway of terrestrial DOM removal and modification in some lakes [54] , and in this context it is important to note that UAL in particular, and FLL are periodically ice covered, whereas LT is not, and thus the exposure time of DOM to ultraviolet also differs between these lakes. Dissolved proteins identified by NMR in FLL during August 2009 could be derived primarily from spring/summer production. However, the fact that the diffusion-edited NMR spectrum of FLL from the previous May (2009) comprised ~50% protein supports the interpretation that at least some of the dissolved proteins are long lived and masked by seasonal terrestrial inputs in late spring. Annual terrestrial SPE-DON inputs into LT from UTR are not sufficient to maintain the calculated SPE-DON inventory of LT ( Supplementary Table 4 ), further supporting a lacustrine source for proteins detected in both LT and FLL. Expectedly, a seasonal signal is absent from UAL because of its small size, absence of winter primary production and short residence time. Radiocarbon signatures of SPE-DOM ( Table 1 ) were compared with potential source isotope signatures to better constrain carbon sources and LT SPE-DOM residence time. The Δ 14 C observations of DIC and DOM in LT ( Table 1 ) cannot be easily reconciled with isotope values of other carbon reservoirs in the region without invoking slow carbon turnover rates in DIC and DOM. In fact, the simple radiocarbon box model suggests an ~60-year residence time for LT DIC in 2009–2010, which translates to a centennial scale residence time for LT SPE-DOM assuming an autochthonous source. This SPE-DOM turnover time is within the estimated replacement time of water in the lake (300–650 years) [34] , [55] , indicating that Δ 14 C observations are consistent with a viable model for inorganic and organic carbon turnover. Together, the radiocarbon model data and NMR spectra support a centennial scale residence time for autochthonous dissolved proteins in LT, where the lake’s exceptionally long residence time exposes the refractory nature of these compounds. With this in mind, the production flux for refractory proteins was calculated and compared with annual atmospheric N loading (148,000 kg; ref. 56 ). Using LT SPE-DOM recoveries and C:N values, the lake’s DON inventory is estimated at ~5 × 10 6 kg N ( Table 1 ; Supplementary Table 4 ). The radiocarbon model suggests this DON reservoir has a 100-year residence time, which translates to an annual production flux of ~50,000 kg N per year for detected proteins, or 34% of the annual incoming atmospheric inorganic N. The SPE-DOM isolated from LT in May 2009 and June 2010 was enriched in 14 C ( Table 1 , Fig. 2 ) compared with January 2010 SPE-DOM from the same location. The enrichment likely results from the mixing together of DOM with distinct endmember Δ 14 C values in a manner similar to what is proposed for marine DOM, which also consists of refractory and ‘fresh’ Δ 14 C endmembers [57] . The proposed mixing model is also consistent with LT’s relatively stable hypolimnion DOC concentration (that is, background) that is seasonally modified by primary production, respiration, small terrestrial inputs and surface mixing ( Supplementary Fig. 2 ). This data set clearly differentiates allochthonous and autochthonous endmembers in the Tahoe basin, and the varying influence of each input can be related to the hydraulic residence time and potential ultraviolet exposure of each lake. The average radiocarbon signature for SPE-DOM from UAL, UTR and to some extent, FLL, together with enriched C:N values and relatively depleted δ 13 C and δ 15 N signatures ( Fig. 2 ), all confirm the terrestrial origin of this DOM. In UAL and seasonally in FLL, the terrestrial influence is prominent because of the small size and shorter water residence time of these lakes ( Supplementary Table 1 ). In contrast, seasonal depletion of C:N, the enrichment of stable isotope signatures, and the prominence of NMR resonances related to proteins together identify autochthonous DOM production in larger lakes (for example, LT), which is likely supported by annual lake mixing that delivers N and P to surface waters ( Supplementary Fig. 9 ). That autochthonous proteins accumulate on long time scales in lakes is a novel finding. The 1 H NMR spectra indicate that biochemicals other than proteins are nearly absent from LT’s SPE-DOM and so, commonly suggested protection mechanisms in soils such as protein encapsulation or modification by glycosylation cannot be important [58] . There are also reports of refractory proteins in marine DOM [59] , [60] ; however, these previous identifications have been indirect and lacked radiocarbon data. There is not enough data to evaluate whether refractory dissolved proteins are prevalent in aquatic environments, but here it is proposed that the combination of photochemical and bacterial degradation of incoming terrestrial DOM, along with low primary production rates in LT, enable the direct detection of these refractory proteins because other types of organic material are nearly absent in LT SPE extracts. These data may have captured a phenomenon restricted to similar lacustrine environments where ultraviolet transparency [51] facilitates photochemical alteration of proteins [61] . Alternatively, retarded degradation of N-rich compounds in this environment may be linked to the limited bioavailability of P 14 , a condition that is prevalent in lake systems and limits LT autotrophy [16] , [62] , [63] and, potentially, heterotrophy [64] . Such limitation on heterotrophic bacteria could make N remineralization less efficient. In summary, the accumulation of dissolved proteins in oligotrophic lakes of the California Sierra Nevada has been definitively identified using a combination of isotope measurements and NMR spectroscopy. The depleted radiocarbon signature of LT SPE-DOM relative to obvious sources suggests that dissolved proteins are selectively preserved. These data further show that autochthonous protein production can sequester as much as 30% of the inorganic N delivered by atmospheric deposition, which is the dominant allochthonous N source to LT (see Supplementary Discussion of potential cultural eutrophication). In the same way that sedimenting particulate organic nitrogen is a sink for inorganic N, the repackaging of N into refractory DON as detected in the Tahoe basin identifies an additional pathway that must be considered when examining mechanisms that impact lake inorganic N:P. Available data on phytoplankton community composition [13] , [65] and regional microbial communities [66] suggest that autochthonous sources of DOM in LT are not unique to this environment. Dissolved organic nitrogen is ubiquitous in aquatic environments and has been previously linked to a variety of processes including grazing of picoplankton and viral lysis, which can release intracellular material rich in protein [67] . Thus, such protein accumulation likely occurs in other systems [9] , [10] , [11] . Data presented here also support the important role of terrestrial organic matter in supporting microbial production in these lakes and thus affecting lake metabolic balance. There is considerable evidence that lake environments will be impacted under future climate change scenarios [12] , [56] . Changes in seasonality and characteristics of hydraulic inputs could alter the quality and quantity of terrestrial organic matter reaching high-elevation lakes, with potential repercussions for DOM cycling as well as ecosystem health. Projections for LT also show that increased stratification will likely reduce nutrient entrainment from depth into surface waters [56] , which may further alter phytoplankton and bacterial community composition. Future investigations of the response of aquatic and terrestrial ecosystems to global change should consider the potential for DOM dynamics to impact nutrient availability and carbon storage. Site description and seasonal sampling Lake water sampling was conducted at LT, FLL, UAL and the UTR. Fallen Leaf Lake is fed by Glen Alpine Creek at its southern end, which drains multiple lakes within the Desolation Wilderness area of the Eldorado National Forest. This lake drains into LT and has a hydraulic lake water residence time of ~8 years ( Fig. 1 and Supplementary Table 1 ). Upper Angora Lake, at the highest elevation of the three lakes sampled, has a water residence times that ranges from <10 days to ~100 days. Sampling was conducted in May/June and August 2009 and January and June/July 2010 to capture seasonal variability in the delivery of allochthonous DOM. Highest stream discharge volumes are typically observed in late spring/early summer during melt-off in the Sierra Nevada ( Supplementary Fig. 1 for UTR), and the majority of allochthonous DOM is likely delivered to lakes during this high flow period. Surface waters of LT were sampled at the TB-4, mid-lake site (water depth of ~440 m), those from FLL were collected at a pier, and UAL and UTR were sampled shore-side ( Fig. 1 ). The UTR was only sampled in July 2010 to determine the source and composition of SPE-DOM entering Lake Tahoe. Lake geochemistry All SPE-DOM samples were collected, filtered and processed on DAX-8 resin according to Aiken et al. [21] with some modifications (see Table 1 for elution solvents). All bulk DOC samples that accompanied SPE-DOM extraction were filtered through combusted 47 mm glass fibre filters (G/FF; Whatman) and collected in combusted glass 40 ml vials ( Table 1 ). Lake Tahoe depth profile and coastal samples were not filtered (that is, TOC; Supplementary Fig. 2 ). The C and N isotopic and elemental content of dried SPE-DOM was assessed using standard elemental analyser isotope ratio mass spectrometry at the Scripps Institution of Oceanography Stable Isotope Facility. Samples for SPE-DOM were not collected at greater depths in LT due to logistical limitations associated with collecting a large volume of water. The fraction of SPE-DOC recovered during extraction and elution was estimated using the dry weight of eluted DOM, measured %C, measured bulk DOC and the total lake-water volume that was filtered ( Table 1 ). This represents the fraction of DOC in each environment that was characterized by the various analyses described here. The 14 C content of DIC and SPE-DOM (including resin and solvent blanks) was determined via accelerator mass spectrometry (AMS) at the National Ocean Sciences AMS (NOSAMS) facility according to established protocols. The Δ 14 C value for the UAL Aug 2009 SPE-DOM sample could not be determined due to problems during sample preparation for 14 C analysis. Samples for DIC were collected before June/July 2010 but are not reported due to sample storage issues. Lignin–phenol analysis followed established protocols [68] , [69] . Further details are provided in the Supplementary Methods . Samples are regularly collected in close proximity to the LT TB-4 collection site and measured for nitrate and chlorophyll concentrations by the UC Davis Tahoe Environmental Research Center [15] , [56] , [70] . NMR spectroscopy Representative samples from all sites were first analysed for their one-dimensional (1D) 1 H NMR spectra at the UCSD-SIO NMR facility (see Supplementary Methods for details). Additional one-dimensional and two-dimensional ( 1 H– 13 C) NMR experiments were conducted on selected samples from LT (June 2010), FLL (May and August of 2009) and UAL (June 2009) at the University of Toronto. These experiments included diffusion editing, STD and HSQC 1 H– 13 C spectroscopy (see Supplementary Methods for details). How to cite this article: Goldberg, S. J. et al. Refractory dissolved organic nitrogen accumulation in high-elevation lakes. Nat. Commun. 6:6347 doi: 10.1038/ncomms7347 (2015).